Cochlear supporting cell transdifferentiation and integration into hair cell layers by inhibition of ephrin-B2 signalling In mammals, cochlear sensory hair cells that are responsible for hearing are postmitotic and are not replaced after loss. One of the most promising strategies to regenerate hair cells is to identify and inhibit the factors preventing the conversion of adjacent non-sensory supporting cells into hair cells. Here we demonstrate that mammalian hair cells can be directly generated from supporting cells by inhibition of ephrin-B2 signalling. Using either ephrin-B2 conditional knockout mice, shRNA-mediated gene silencing or soluble inhibitors, we found that downregulation of ephrin-B2 signalling at embryonic stages results in supporting cell translocation into hair cell layers and subsequent switch in cell identity from supporting cell to hair cell fate. As transdifferentiation is here a result of displacement across boundary, this original finding presents the interest that newly generated hair cells directly integrate either hair cell layer, then would be likely more rapidly able to fit into functional circuitry. In mammals, sounds are perceived through mechanosensory hair cells located within the sensory epithelium of the cochlea (the organ of Corti). Hair cells produced during development are postmitotic and are not replaced after loss [1] , [2] , [3] , [4] . As a result, deafness due to hair cell loss is irreversible. Hair cells and adjacent supporting cells arise from a common progenitor that acquires a hair cell or supporting cell phenotype via lateral inhibition mediated by the Notch signalling pathway [3] , [5] , [6] . One of the most promising strategies to regenerate hair cells is to identify and inhibit the factors preventing the conversion of supporting cells into hair cells. For instance, it is well known that supporting cells are prevented from differentiating into hair cells through Notch signalling triggered by ligands expressed by adjacent hair cells [6] , [7] . Taking advantage of this observation, it has been shown recently that Notch inhibition induces cochlear hair cell regeneration and recovery of hearing after acoustic trauma [8] . Within the organ of Corti, hair cells and several types of specialized supporting cells are organized in a regular mosaic pattern that extends along the basal-to-apical axis of the cochlear duct. One of the most striking aspects of this mosaic is that specific cell types are arranged in discrete rows. The edge of the organ of Corti located closest to the modiolus (modiolar boundary) is composed of a single row of alternating inner hair cells and border/inner phalangeal cells ( Fig. 1a ). Directly adjacent to the inner hair cell row are two rows of pillar cells. Then, three or four rows of outer hair cells and Deiters’ cells are also arranged into a regular alternating mosaic. Finally, the edge of the organ of Corti located closest to the stria vascularis (strial boundary) is formed by the interface between the most strial row of outer hair cells and directly adjacent Hensen’s cells. How hair cells and supporting cells are maintained in distinct rows and compartments still remains unknown. 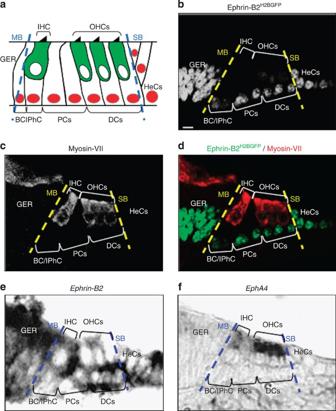Figure 1: Ephrin-B2 and EphA4 display complementary expression patterns in the developing organ of Corti. (a) Schematic representation of cell patterning in the organ of Corti. Between the modiolar (MB) and strial (SB) boundaries, myosin-VII+inner (IHC) and outer hair cells (OHCs, green) and p27kip1+supporting cells (red) are organized in alternating rows. Beyond the strial boundary are p27kip1+Hensen’s cells (HeCs). (b–d) Representative example of myosin-VII immunolabelling on transversal section of an E16ephrin-B2+/H2BGFPorgan of Corti showing that ephrin-B2H2BGFPexpression is restricted to both supporting cells and greater epithelial ridge (GER). (e,f) Representative example ofin situhybridization on transversal sections of an E16 organ of Corti showing thatephrin-B2expression is restricted to both supporting cells and GER (e), whereasEphA4expression is specifically restricted to hair cells (f), thereby displaying complementary expression patterns. Each of these expression patterns was observed on over ten sections. Scale bar inbrepresents 5 μm inb–f. BC, border cell; DCs, Deiters’ cells; IPhC, inner phalangeal cell; PCs, pillar cells. Figure 1: Ephrin-B2 and EphA4 display complementary expression patterns in the developing organ of Corti. ( a ) Schematic representation of cell patterning in the organ of Corti. Between the modiolar (MB) and strial (SB) boundaries, myosin-VII + inner (IHC) and outer hair cells (OHCs, green) and p27kip1 + supporting cells (red) are organized in alternating rows. Beyond the strial boundary are p27kip1 + Hensen’s cells (HeCs). ( b – d ) Representative example of myosin-VII immunolabelling on transversal section of an E16 ephrin-B2 +/H2BGFP organ of Corti showing that ephrin-B2 H2BGFP expression is restricted to both supporting cells and greater epithelial ridge (GER). ( e , f ) Representative example of in situ hybridization on transversal sections of an E16 organ of Corti showing that ephrin-B2 expression is restricted to both supporting cells and GER ( e ), whereas EphA4 expression is specifically restricted to hair cells ( f ), thereby displaying complementary expression patterns. Each of these expression patterns was observed on over ten sections. Scale bar in b represents 5 μm in b – f . BC, border cell; DCs, Deiters’ cells; IPhC, inner phalangeal cell; PCs, pillar cells. Full size image Among gene families that have been shown to control tissue morphogenesis, ephrins and their Eph receptors are good candidates for patterning different cell types in the organ of Corti. This large Eph family has been classified into two subclasses, EphA and EphB, according to their affinity for either glycosylphosphatidylinositol-anchored ephrin-A or transmembrane ephrin-B ligands [9] . Based on its well-described role in boundary formation between adjacent cell types by interacting with specific EphA4 or EphB receptors [10] , [11] , [12] , [13] , [14] , we suggested ephrin-B2 to be involved in a repulsive system allowing cell sorting across the hair cell/supporting cell interface in the organ of Corti. As it has been proposed that cells that can migrate across non-lineage boundaries switch their phenotype to adapt to the identity of their local neighbours [15] , [16] , [17] , manipulating these boundaries could represent an unexpected strategy to generate additional hair cells. Here we demonstrate that hair cells can be directly generated from supporting cells by inhibition of ephrin-B2 signalling. Using either ephrin-B2 conditional knockout mice, short hairpin RNA (shRNA)-mediated gene silencing or soluble inhibitors, we found that downregulation of ephrin-B2 signalling at late embryonic stages, that is, after the normal period of hair cell production, results in supporting cell translocation into hair cell layers and subsequent switch in cell identity from supporting cell to hair cell fate. Supporting cell-specific expression of ephrin-B2 To test whether ephrin-B2 forms a gene-expression boundary at the hair cell/supporting cell interface, we first analysed GFP expression in the organ of Corti of an ephrin-B2 +/H2BGFP mouse model, in which a nuclear GFP gene, H2BGFP , has been knocked into the Efnb2 locus [18] . GFP labelling was found to be specifically restricted to both supporting cells and greater epithelial ridge from embryonic day (E) 16, that is, as soon as distinct hair cell morphologies begin to be apparent [19] ( Fig. 1b–d ). Such expression profile distinguishing hair cells from adjacent supporting cells persists in the post-hearing-onset cochlea ( Supplementary Fig. 1 ) and was further confirmed by in situ hybridization ( Fig. 1e ). In the same aforementioned embryonic time window, we found that, among Eph receptors that are known to interact with ephrin-B2 (EphA4 end EphBs), EphA4 was the only one to be exclusively expressed in both inner and outer hair cells in agreement with previous observations [20] , [21] ( Fig. 1f and Supplementary Fig. 2 ). These data, therefore, suggest that ephrin-B2 and EphA4 display complementary expression patterns in the developing organ of Corti, consistent with a role in cell sorting across the hair cell/supporting cell interface. Interestingly, both of these proteins were found to be required for hearing function [22] , [23] . Supporting cell transdifferentiation by loss of ephrin-B2 To test whether in vivo inhibition of ephrin-B2 can be proposed as a strategy to produce extra hair cells, we used a mouse model in which ephrin-B2 is conditionally deleted from glial fibrillary acidic protein-expressing supporting cells [24] , [25] , that is, in all supporting cells that are directly in contact with hair cells [26] , [27] ( Supplementary Fig. 3 ). Using parvalbumin labelling as a hair cell-specific marker [28] , we found that GFAP +/cre ;ephrin-B2 lox/lox newborn mice exhibit a significant increase in extra inner and outer hair cells compared with WT mice ( Fig. 2a,b,i ). Importantly, these cells appear not to be produced randomly but rather arise contiguously to pre-existing hair cells and thereby integrate either inner or outer hair cell layer. To know whether extra hair cells come from direct supporting cell transdifferentiation, we used an additional sox2 supporting cell-specific marker [19] , [29] . Whereas parvalbumin and sox2 are usually restricted to hair cell and supporting cell populations in neonatal cochleae, respectively, we observed a significant increase in parvalbumin + /sox2 + cells in GFAP +/cre ;ephrin-B2 lox/lox mice compared with WT animals ( Fig. 2c–h,j ), meaning that extra hair cells come from direct transdifferentiation of supporting cells. These cells develop stereocilia and are targets of innervation, suggesting a functional integration in the sensorineural circuitry ( Supplementary Fig. 4 ). 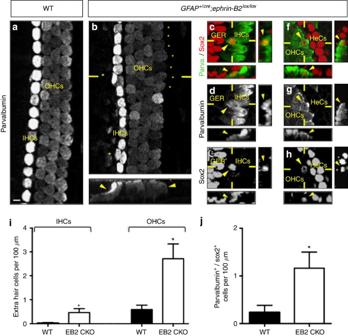Figure 2:In vivoloss of ephrin-B2 induces supporting cells to transdifferentiate into inner and outer hair cells. Parvalbumin immunolabelling alone (a,b) or in combination with sox2 (c–h) of whole-mount cochleae from newborn WT (a) andGFAP+/cre;ephrin-B2lox/loxmice (b–h). Extra inner (IHCs) and outer hair cells (OHCs) arise contiguously to pre-existing hair cells in the absence ofephrin-B2(asterisks and arrowheads inb). Some of these extra IHCs (c–e) and OHCs (f–h) are positive for both parvalbumin and sox2 (arrowheads). The number of extra IHCs and OHCs (i) and the number of parvalbumin+/sox2+cells per 100 μm of whole-mount cochlea (j) is significantly increased inGFAP+/cre;ephrin-B2lox/lox(EB2 CKO) compared with WT mice (n=4 animals per genotype; *P=0.0372 for IHCs, *P=0.0171 for OHCs, *P=0.0458 for parvalbumin+/sox2+cells). Statistical significance was determined using a Student’st-test. Data are presented as mean±s.e.m. Scale bar inarepresents 5 μm ina–h. GER=greater epithelial ridge, HeCs=Hensen’s cells. Figure 2: In vivo loss of ephrin-B2 induces supporting cells to transdifferentiate into inner and outer hair cells. Parvalbumin immunolabelling alone ( a , b ) or in combination with sox2 ( c – h ) of whole-mount cochleae from newborn WT ( a ) and GFAP +/cre ;ephrin-B2 lox/lox mice ( b – h ). Extra inner (IHCs) and outer hair cells (OHCs) arise contiguously to pre-existing hair cells in the absence of ephrin-B2 (asterisks and arrowheads in b ). Some of these extra IHCs ( c – e ) and OHCs ( f – h ) are positive for both parvalbumin and sox2 (arrowheads). The number of extra IHCs and OHCs ( i ) and the number of parvalbumin + /sox2 + cells per 100 μm of whole-mount cochlea ( j ) is significantly increased in GFAP +/cre ;ephrin-B2 lox/lox (EB2 CKO) compared with WT mice ( n =4 animals per genotype; * P =0.0372 for IHCs, * P =0.0171 for OHCs, * P =0.0458 for parvalbumin + /sox2 + cells). Statistical significance was determined using a Student’s t -test. Data are presented as mean±s.e.m. Scale bar in a represents 5 μm in a – h . GER=greater epithelial ridge, HeCs=Hensen’s cells. Full size image Ex vivo transdifferentiation by mosaic ephrin-B2 silencing At boundaries, loss of an ephrin-B gene expression in a mosaic of cells may cause more severe defects than loss of expression in all cells [30] , [31] , [32] . This is because the differential ephrin-B expression makes cells that should be the same behave as distinct populations, whereas they remain a homogenous population if all the cells lack ephrin-B expression [30] , [31] , [32] , [33] . We then further examined the effect of acute ephrin-B2 silencing at a single supporting cell-scale (thereby artificially creating a mosaic loss of ephrin-B2 signalling at the hair cell/supporting cell interface) by using shRNA electroporation in E16 cochleae. Four ephrin-B2-specific and one irrelevant short interfering RNAs (siRNAs) were initially transfected in N2A cells and their protein knockdown efficiency was assessed by western blotting ( Fig. 3a and Supplementary Fig. 5 ). Two of them were selected, annealed and subcloned into pCA-b-EGFPm5 silencer 3 vector [34] and one of these two constructs provided an efficient in situ downregulation of ephrin-B2 expression ( Fig. 3b–e ) without increasing cell death ( Supplementary Fig. 6 ). We used myosin-VII as a marker of hair cells [35] and p27 kip1 as a specific nuclear marker of supporting cells [36] , [37] . As expected, hair cells or supporting cells transfected with scrambled shRNA were found to express their own and unique specific marker, that is, myosin-VII or p27 kip1 , respectively ( Fig. 3f–i ). By contrast, when targeted by the specific ephrin-B2 shRNA, some cells located on the hair cell side of the hair cell/supporting cell boundary revealed an intermediate identity, by simultaneously expressing p27 kip1 and myosin-VII ( Fig. 3k–n and Supplementary Fig. 7 ). The percentage of EGFP + /p27 kip1+ /myosin-VII + cells among the total amount of EGFP + /p27 kip1+ cells present at the hair cell/supporting cell interface was significantly increased when using ephrin-B2 shRNA compared with scrambled shRNA ( Fig. 3j and Supplementary Fig. 8 ). Importantly, these EGFP + /p27 kip1+ /myosin-VII + cells appear to be less p2 7kip1+ than most of the supporting cells directly located on the supporting cell side of the hair cell/supporting cell boundary (compare yellow and white arrowheads on Fig. 3l,m ), suggesting a transient phenotype while translocating from the supporting cell to the hair cell layer. As myosin-VII + hair cells are never positive for p27 kip (refs 11 , 36 , 37 ), such co-expression of myosin-VII and p27 kip1 unambiguously means that EGFP + /p27 kip1+ cells moved from the supporting cell compartment towards the hair cell layer because of loss of ephrin-B2 expression and, as a consequence, progressively switch their identity. Indeed, a sudden cell-autonomous overexpression of p27 kip1 in a pre-existing hair cell due to an shRNA-mediated ephrin-B2 silencing would be rather unlikely given that hair cells do not express ephrin-B2. Importantly, it should be noticed that transfected supporting cells that do not translocate in the hair cell layer do not change their fate, meaning that cell displacement is a necessary condition for transdifferentiation ( Supplementary Fig. 9 ). 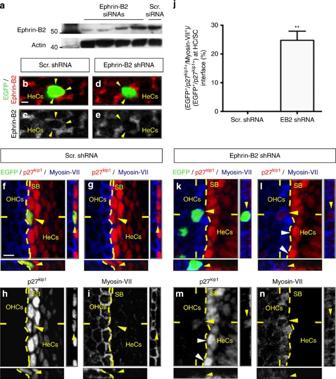Figure 3: Ephrin-B2 expression silencing induces supporting cell translocation into the hair cell layer and transdifferentiation. Ex vivoelectroporation of E16 cochleae using Enhanced green fluorescent protein control (f–i) or targeted shRNA construct againstephrin-B2transcript (k–n). (a) Assessment of ephrin-B2 siRNAs knockdown efficiency using western blotting. (b–e)In situassessment of ephrin-B2 shRNA knockdown efficiency after electroporation using ephrin-B2 immunolabelling focused in the Hensen’s cells (HeCs) layer. EGFP overlaps with ephrin-B2 labelling when using scrambled (Scr.) shRNA (arrowheads inb,c), whereas it does not when using ephrin-B2-targeted shRNA (arrowheads ind,e). (f–i,k–n) Double immunolabelling for p27kip1and myosin-VII. (f–i) Representative example of an EGFP-labelled p27kip1+supporting cell transfected using control shRNA and staying in the supporting cell compartment (arrowhead). (j) The percentage of EGFP+/p27kip1+/myosin-VII+among the total amount of EGFP+/p27kip1+cells at the hair cell/supporting cell interface is significantly increased when using ephrin-B2 shRNA compared with Scr. shRNA (n=3 independent experiments for each condition; **P=0.0014). Statistical significance was determined using a Student’st-test. Data are presented as mean±s.e.m. (k–n) Representative example of an EGFP-labelled p27kip1+/myosin-VII+cell transfected with an ephrin-B2 shRNA (yellow arrowhead) located in the hair cell side of the strial boundary (SB, dotted curve). Note that such EGFP+/p27kip1+/myosin-VII+cell appears to be less p27kip1+(yellow arrowhead) than most of the supporting cells directly located on the supporting cell side of the SB (white arrowheads) suggesting an intermediate phenotype while switching from supporting cell to hair cell fate. Scale bar inbrepresents 2 μm inb–eand in (f) represents 5 μm in (f–i,k–n). OHCs=outer hair cells. Figure 3: Ephrin-B2 expression silencing induces supporting cell translocation into the hair cell layer and transdifferentiation. Ex vivo electroporation of E16 cochleae using Enhanced green fluorescent protein control ( f – i ) or targeted shRNA construct against ephrin-B2 transcript ( k – n ). ( a ) Assessment of ephrin-B2 siRNAs knockdown efficiency using western blotting. ( b – e ) In situ assessment of ephrin-B2 shRNA knockdown efficiency after electroporation using ephrin-B2 immunolabelling focused in the Hensen’s cells (HeCs) layer. EGFP overlaps with ephrin-B2 labelling when using scrambled (Scr.) shRNA (arrowheads in b , c ), whereas it does not when using ephrin-B2-targeted shRNA (arrowheads in d , e ). ( f – i , k – n ) Double immunolabelling for p27 kip1 and myosin-VII. ( f – i ) Representative example of an EGFP-labelled p27 kip1+ supporting cell transfected using control shRNA and staying in the supporting cell compartment (arrowhead). ( j ) The percentage of EGFP + /p27 kip1+ /myosin-VII + among the total amount of EGFP + /p27 kip1+ cells at the hair cell/supporting cell interface is significantly increased when using ephrin-B2 shRNA compared with Scr. shRNA ( n =3 independent experiments for each condition; ** P =0.0014). Statistical significance was determined using a Student’s t -test. Data are presented as mean±s.e.m. ( k – n ) Representative example of an EGFP-labelled p27 kip1+ /myosin-VII + cell transfected with an ephrin-B2 shRNA (yellow arrowhead) located in the hair cell side of the strial boundary (SB, dotted curve). Note that such EGFP + /p27 kip1+ /myosin-VII + cell appears to be less p27 kip1+ (yellow arrowhead) than most of the supporting cells directly located on the supporting cell side of the SB (white arrowheads) suggesting an intermediate phenotype while switching from supporting cell to hair cell fate. Scale bar in b represents 2 μm in b – e and in ( f ) represents 5 μm in ( f – i , k – n ). OHCs=outer hair cells. Full size image Switch in supporting cell identity by ephrin-B2 inhibition To further confirm that adjacent supporting cells can really be reprogrammed into hair cells when disrupting ephrin-B2 signalling, we designed an organotypic assay in which explants of organ of Corti isolated from E16 cochleae were cultured for 4 days in the presence of control IgG-Fc or EphA4-Fc, a soluble inhibitor known to have a high affinity for ephrin-B2 (refs 9 , 38 ). In control condition, the organ of Corti exhibit sharp boundaries with cells displaying a clear and unique phenotype (myosin-VII or p27 kip1 /sox2), as expected ( Fig. 4a–d ). By contrast, when blocking ephrin-B2 signalling, a subset of cells become simultaneously positive for p27 kip1 , sox2 and myosin-VII, unambiguously revealing an intermediate and switching phenotype, especially both at the strial (between outer hair cells and Hensen’s cells, Fig. 4e–h ) and modiolar (within or very close to the row of inner hair cells, Fig. 4i–l ) boundaries of the organ of Corti. The number of these myosin-VII + /p27 kip1+ /sox2 + cells is significantly higher in EphA4-Fc compared with control condition ( Fig. 4m ). Interestingly, among the same cell population, myosin-VII and p27 kip1 display opposing gradients of expression that are perpendicular to the strial boundary of the organ of Corti, suggesting a typical behaviour of cells that are progressively changing their own identity. As a consequence, myosin-VII + /p27 kip1+ /sox2 + cells appear to be less p27 kip1+ than supporting cells but more than hair cells (p27 kip1+ supporting cells>p27 kip1+/− supporting cells/hair cells (arrowheads on magnification of Fig. 4g ) >p27 kip1− hair cells) and simultaneously more myosin-VII + than supporting cells but less than hair cells (myosin-VII − supporting cells<myosin-VII +/− supporting cells/hair cells (arrowheads on magnification of Fig. 4f )<myosin-VII + hair cells). This striking feature is exemplified by the difficulty to segregate myosin-VII + hair cell from p27 kip1+ supporting cell populations at both strial (dotted curve on magnifications of Fig. 4e–g ) and modiolar (dotted line on Fig. 4i–k ) boundaries, as can be easily realized in control condition (dotted line on Fig. 4a–c ). Importantly, the supporting cells that are not in contact with hair cells never co-express p27 kip1 , myosin-VII and sox2. Indeed, cells with a mixed identity are exclusively located within either inner or outer hair cell layer or arise contiguously to pre-existing hair cells, suggesting that cell displacement is required for transdifferentiation. These results seem to faithfully reproduce those obtained using shRNA electroporations, showing evidence that inhibition of ephrin-B2 signalling results in supporting cell translocation into hair cell layers and subsequent transdifferentiation. Similar results were obtained using an ephrin-B2-Fc inhibitor, reinforcing the idea that an ephrin-B2/EphA4-EphB signalling acts to segregate hair cells from supporting cells ( Supplementary Fig. 10 ). However, either using shRNA-mediated gene silencing or soluble inhibitors, since translocating cells progressively lose the supporting cell marker p27 kip1 while switching their own phenotype, it is likely that our results underestimate the rate of transdifferentiated cells due to the fraction of the latter cells that finally become undetectable. For instance, it appears that transdifferentiating supporting cells lose rapidly p27 kip1 expression as they invade the hair cell layer but remain longer positive for sox2 ( Fig. 4e,h,n and Supplementary Fig. 10 ), in agreement with the fact that sox2 is likely required for transdifferentiation of supporting cells to hair cells during regeneration [39] . 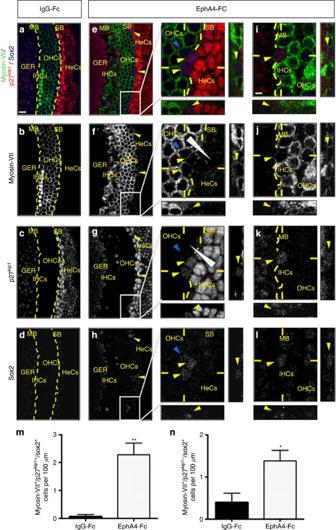Figure 4: Blocking ephrin-B2 signalling results in supporting cell integration into either hair cell layer and switch in cell identity. In vitroorganotypic assay using organs of Corti cultured in the presence of control (IgG-Fc,a–d) or soluble inhibitor EphA4-Fc (e–l) reagents. Triple immunolabelling for myosin-VII, p27kip1and sox2. (a–d) In control condition, the organ of Corti exhibits sharp boundaries (dotted line ina–c) with cells displaying a clear and unique phenotype (myosin-VII+or p27kip1+). (e–l) When blocking ephrin-B2 signalling, a subset of cells (yellow arrowheads) become simultaneously positive for myosin-VII, p27kip1and sox2, both at the strial (SB) (e–hand magnifications) and modiolar (MB) boundaries (i–l). Myosin-VII and p27kip1display opposite gradients of expression that are perpendicular to the SB (triangular shape on magnifications off,g). Myosin-VII+hair cell and p27kip1+supporting cell populations cannot be easily segregated along either SB or MB (dotted curve on magnifications ofe–gandi–k). As transdifferentiating myosin-VII+/p27kip1+/sox2+supporting cells (yellow arrowheads on magnifications ofe–h) translocate into the hair cell layer, these cells reinforce their expression in myosin-VII while losing p27kip1expression but remain longer positive for sox2 (blue arrowhead on magnifications ofe–h). (m,n) The number of either myosin-VII+/p27kip1+/sox2+or myosin-VII+/p27kip1−/sox2+cells per 100 μm of explant is significantly increased in the presence of EphA4-Fc compared with control condition (n=3 independent experiments for each condition; **P=0.0064 for myosin-VII+/p27kip1+/sox2+cells, *P=0.0362 for myosin-VII+/p27kip1−/sox2+cells). Statistical significance was determined using Student’st-test. Data are presented as mean±s.e.m. Scale bar inarepresents 10 μm ina–hand inirepresents 2 μm ini–l. GER, greater epithelial ridge; HeCs, Hensen’s cells; IHCs, inner hair cells; OHCs, outer hair cells. Figure 4: Blocking ephrin-B2 signalling results in supporting cell integration into either hair cell layer and switch in cell identity. In vitro organotypic assay using organs of Corti cultured in the presence of control (IgG-Fc, a – d ) or soluble inhibitor EphA4-Fc ( e – l ) reagents. Triple immunolabelling for myosin-VII, p27 kip1 and sox2. ( a – d ) In control condition, the organ of Corti exhibits sharp boundaries (dotted line in a – c ) with cells displaying a clear and unique phenotype (myosin-VII + or p27 kip1+ ). ( e – l ) When blocking ephrin-B2 signalling, a subset of cells (yellow arrowheads) become simultaneously positive for myosin-VII, p27 kip1 and sox2, both at the strial (SB) ( e – h and magnifications) and modiolar (MB) boundaries ( i – l ). Myosin-VII and p27 kip1 display opposite gradients of expression that are perpendicular to the SB (triangular shape on magnifications of f , g ). Myosin-VII + hair cell and p27 kip1+ supporting cell populations cannot be easily segregated along either SB or MB (dotted curve on magnifications of e – g and i – k ). As transdifferentiating myosin-VII + /p27 kip1+ /sox2 + supporting cells (yellow arrowheads on magnifications of e – h ) translocate into the hair cell layer, these cells reinforce their expression in myosin-VII while losing p27 kip1 expression but remain longer positive for sox2 (blue arrowhead on magnifications of e – h ). ( m , n ) The number of either myosin-VII + /p27 kip1+ /sox2 + or myosin-VII + /p27 kip1− /sox2 + cells per 100 μm of explant is significantly increased in the presence of EphA4-Fc compared with control condition ( n =3 independent experiments for each condition; ** P =0.0064 for myosin-VII + /p27 kip1+ /sox2 + cells, * P =0.0362 for myosin-VII + /p27 kip1− /sox2 + cells). Statistical significance was determined using Student’s t -test. Data are presented as mean±s.e.m. Scale bar in a represents 10 μm in a – h and in i represents 2 μm in i – l . GER, greater epithelial ridge; HeCs, Hensen’s cells; IHCs, inner hair cells; OHCs, outer hair cells. Full size image Here we demonstrate that manipulation of an ephrin gene expression boundary at early stages could be used as a new strategy for directly changing supporting cells into hair cells in the cochlea. We observed that disruption of ephrin-B2 signalling results in supporting cell translocation into hair cell layers and, in agreement with previous models about mechanisms of non-lineage boundary formation, switch in cell identity [15] , [16] , [17] ( Fig. 5b,c ). This finding is also consistent with the fact that mammalian cochlear supporting cells can divide and transdifferentiate into hair cells [36] . Importantly, such change in cell fate exclusively occurs at the interface between hair cells and supporting cells, reinforcing the idea that transdifferentiation is a consequence of local inhibition of ephrin-B2 signalling-mediated hair cell/supporting cell boundary. In this context, it is reasonable to wonder why supporting cells can transdifferentiate into hair cells and not the other way around. A possible explanation could be that supporting cells but not hair cells maintain sox2 expression, a transcription factor known to be required for transdifferentiation of supporting cells into hair cells during regeneration [39] . Nevertheless, how such cell fate change precisely occurs remains unclear. Interestingly, however, our results suggest that ephrin-B2 and Notch are expressed in similar supporting cell types throughout the development [6] . Therefore, as shown during vasculogenesis [40] , [41] , ephrin-B2 could be a downstream target of Notch signalling in supporting cells required to segregate the latter cells from adjacent hair cells. In support of this hypothesis, it was proposed that Notch signalling couples cell segregation and differentiation at hindbrain boundaries [42] , [43] . As a consequence, loss of a Notch pathway component could weaken the supporting cell fate and make easier the switch towards the hair cell phenotype. In normal condition, it is therefore likely that ephrin-B2 from supporting cells interacts with at least one of its specific receptors expressed by hair cells, such as EphA4 to maintain hair cells and supporting cells in distinct rows and compartments ( Fig. 5a ). 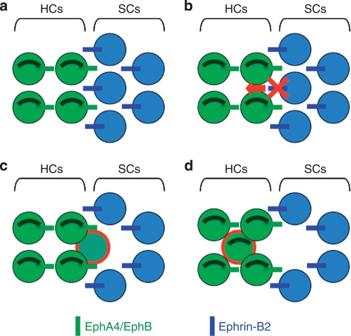Figure 5: A model for how inhibition of ephrin-B2 signalling induces supporting cell translocation into the hair cell layer and transdifferentiation. (a) Ephrin-B2 signalling maintains hair cells (HCs) and supporting cells (SCs) in distinct rows and compartments. (b,c) Mosaic ephrin-B2 silencing at the hair cell/supporting cell interface allows supporting cell to translocate into the hair cell layer while switching from supporting cell to hair cell fate (circled in red inc). (d) The former supporting cell has completely integrated the hair cell layer, lost supporting cell markers and become a fully differentiated hair cell (circled in red). Figure 5: A model for how inhibition of ephrin-B2 signalling induces supporting cell translocation into the hair cell layer and transdifferentiation. ( a ) Ephrin-B2 signalling maintains hair cells (HCs) and supporting cells (SCs) in distinct rows and compartments. ( b , c ) Mosaic ephrin-B2 silencing at the hair cell/supporting cell interface allows supporting cell to translocate into the hair cell layer while switching from supporting cell to hair cell fate (circled in red in c ). ( d ) The former supporting cell has completely integrated the hair cell layer, lost supporting cell markers and become a fully differentiated hair cell (circled in red). Full size image Altogether, our results identified a new unexpected mechanism to directly convert supporting cell fate into hair cell fate. Interestingly, the fact that ephrin-B2 expression distinguishing hair cells from adjacent supporting cells persists in the post-hearing-onset cochlea could lead to strategies aimed at regenerating the sensory epithelium after partial or complete loss of hair cells. Beside most classical approaches showing that hair cells can be generated at random ectopic positions by Math1 overexpression [44] , [45] , [46] , such original strategy alternatively offers the advantage that newly generated hair cells directly integrate either hair cell layer ( Fig. 5d ), then would be likely more rapidly able to participate in functional circuitry. Animals Ephrin-B2 +/H2BGFP mice were generated as described [18] . GFAP +/cre ;ephrin-B2 lox/lox newborn mice were obtained from breeding of GFAP +/cre 24 with ephrin-B2 lox/lox mice [25] . Mice were group-housed in the animal facility of the University of Liège under standard conditions with food and water ad libitum and were maintained on a 12-h light/dark cycle. All animals were taken care in accordance with the Declaration of Helsinki and following the guidelines of the Belgian ministry of agriculture in agreement with EC laboratory animal care and use regulation (86/609/CEE, CE of J n°L358, 18 December 1986). RNA in situ hybridization In situ hybridization was performed using digoxigenin-labelled ephrin-B2 , EphA4 , EphB1 , EphB2 and EphB3 riboprobes [10] , [47] , [48] as previously described [49] . Sections were air-dried, washed in PBS and post-fixed in paraformaldehyde. After treatment with 100 m M triethanolamine, pH 8, acetylated (by adding dropwise acetic anhydride 0.25%) while rocking 15 min at room temperature (RT), slides were washed three times in PBS-0.1% Tween-20 and pre-hybridized in pre-warmed hybridization cocktail 50% formamide (Amresco) at least 60 min at 70 °C. Afterwards, sections were hybridized with 800 ng ml −1 RNA probes overnight at 70 °C. Sections were then washed twice in pre-warmed washing buffer (50% formamide, 2 × sodium salt citrate, 0.1% Tween-20) for 60 min at 70 °C. Slides were pre-incubated for 1 h in blocking solution (Tris-Saline buffer (100 mM Tris pH 7.5; 150 mM NaCl) containing 10% Normal Goat Serum (Dako)) at RT and subsequently incubated overnight at 4 °C with anti-digoxigenin antibody coupled to alkaline phosphatase (1:2,000, Roche Applied Science) diluted in blocking solution. After three washes with Tris-Saline buffer, sections were finally overlaid with 200 μl filtered NBT/BCIP (Nitro Blue Tetrazolium/5-Bromo-4-Chloro-3-Indolyl Phosphate) −0.1% Tween-20 solution (Sigma-Aldrich) between coverslips in dark and at RT until the signal appears. Slides were then washed, post-fixed and mounted in aquamount medium (BDH laboratories). ShRNA-expressing constructs and electroporation Four purified target siRNA duplexes directed against distinct sites in the ephrin-B2 transcript (designed by Dharmacon RNAi Technologies) and one irrelevant siRNA were transfected into N2A cells using Lipofectamine reagent (Invitrogen) and further cultured for 48 h. To assess the knockdown efficiency, proteins were isolated and analysed by western blotting using ephrin-B2 antibody (rabbit IgG, 1:500, Santa Cruz Biotechnology). Bands were compared at expected molecular weight of 55 kDa (ref. 50 ; Supplementary Fig. 5 ). Based on these results, the two following sequences were then annealed and subcloned into modified pCA-b-EGFPm5 silencer 3 vector [34] —ephrin-B2 siRNA 01, 5′-CCAAAUUUCUACCCGGACA-3′ and ephrin-B2 siRNA 02, 5′-GCAUAUUUGUGCCGUAAUU-3′. Primers for sequencing were purchased from Eurogentec SA. In situ knockdown efficiency of shRNAs was assessed using ephrin-B2 antibody (goat IgG, 1:100, R&D Systems) after electroporation. Cochleae were dissected from E16 mice, transferred in a sterile Petri dish and injected at the apex with a solution containing 2 μg μl −1 of plasmid DNA, PBS-10% glucose and Fast-Green (Sigma-Aldrich) using pulled borosilicate needles and Femtojet microinjector (VWR). Before electroporation, the central axis of the cochlea was carefully oriented perpendicular to the electrodes (Sonidel). Eight electrical pulses were then applied at 30 V (50 ms duration) with 500 ms intervals using ECM-830 BTX square wave electroporator (BTX, Gentronic). Explants were dissected and cultured for 4 days. Tissues were then fixed in 4% Paraformaldehyde, washed in PBS and immunolabelled. In vitro organotypic assay Organs of Corti were isolated from E16 mouse cochleae and cultured onto Millicell Culture Insert (Millipore) in DMEM (Gibco) supplemented with glucose (final concentration 6 g l −1 ) and N1 additives (insulin (5 μg ml −1 ) transferrin (5 μg ml −1 putrescin (10 −4 M), progesterone (2 × 10 −8 M) and selenium ((Na 2 SeO 3 ) 3 × 10 −8 M)). Explants were treated with either IgG-Fc fragment as control, recombinant mouse EphA4-Fc or ephrin-B2-Fc chimera (20 μg ml −1 ; R&D Systems), during 4 days. Tissue processing and immunostainings Sections, whole-mount cochleae or explants were incubated overnight at 4 °C with primary antibodies directed against GFP (rabbit IgG, 1:200; Torrey Pines Biolabs), parvalbumin (mouse IgG1, clone PARV-19, 1:250; Sigma-Aldrich), myosin-VII (rabbit IgG, 1:250; Santa Cruz Biotechnology), p27 kip1 (mouse IgG1, 1:250; BD Biosciences), sox2 (goat IgG, 1:250; Santa Cruz Biotechnology), active caspase-3 (rabbit IgG, 1:250; Promega) or neurofilament H (rat IgG, clone TA51, 1:1,000; Millipore). Fluorescein isothiocyanate-phalloidin (1:500; Sigma-Aldrich) was used as an F-actin marker. Tissues were then incubated for 1 h with either Rhodamine Red X-, FITC- or Cy5-conjugated goat anti-mouse, anti-rabbit or anti-rat IgGs secondary antibodies (Jackson Immunoresearch Laboratories). Confocal microscopy, image analysis and quantification Confocal fluorescence images were acquired using the Olympus Fluoview FV1000 confocal system (Olympus Europa GmbH). Unless otherwise mentioned, fields were acquired using Z-scan, with a step of 0.5 μm between each confocal plane in order to create orthogonal projections when needed. For comparison between culture conditions, all preparations were analysed at the same time, using the same acquisition parameters. To compare the number of parvalbumin + extra inner and outer hair cells and the number of parvalbumin + /sox2 + hair cells on whole-mount cochleae from newborn WT and GFAP +/cre ;ephrin-B2 lox/lox mice, three regions measuring at least 300 μm and corresponding to apical, middle and basal turns of the cochlea were considered for quantification. Values were expressed as a mean number of cells per 100 μm. Data were statistically analysed using a Student’s t -test. P- values <0.05 were considered significant (* P <0.05). To assess the proportion of transfected supporting cells that are believed displaced towards the hair cell compartment, we only considered supporting cells directly adjacent to hair cells. We evaluated the percentage of EGFP + /p27 kip1+ /myosin-VII + cells among the total amount of EGFP + /p27kip1 + at the hair cell/supporting cell interface. EGFP + cells were considered transdifferentiating when at least half of the p27kip1 + nucleus was surrounded by myosin-VII + labelling in the three axes. For each transfection, all the EGFP + /p27kip1 + cells observed at the hair cell/supporting cell interface were considered for the statistical analysis. Each statistical value represents a mean of three independent experiments ( Supplementary Fig. S6 ). Data were statistically analysed using a Student’s t -test. P- value <0.05 was considered significant (** P <0.01). For each control IgG-Fc, EphA4-Fc or ephrin-B2-Fc condition, we quantified and compared the number of myosin-VII + /p27 kip1+ /sox2 + and myosin-VII + /p27 kip1− /sox2 + cells in explants after 4 days in culture. Three regions measuring at least 300 μm and corresponding to apical, middle and basal turns of the cochlea were taken into account for quantification. Cells were considered transdifferentiating when at least half of the p27kip1 + and/or sox2 + nucleus was surrounded by myosin-VII + labelling in the three axes. Values were expressed as a mean number of cells per 100 μm. Each statistical value represents a mean of three independent experiments. Data were statistically analysed using a Student’s t -test. P- values <0.05 were considered significant (* P <0.05; ** P <0.01). How to cite this article : Defourny, J. et al. Cochlear supporting cell transdifferentiation and integration into hair cell layers by inhibition of ephrin-B2 signalling. Nat. Commun. 6:7017 doi: 10.1038/ncomms8017 (2015).